Structural characterization of tin in toothpaste by dynamic nuclear polarization enhanced119Sn solid-state NMR spectroscopy Stannous fluoride (SnF 2 ) is an effective fluoride source and antimicrobial agent that is widely used in commercial toothpaste formulations. The antimicrobial activity of SnF 2 is partly attributed to the presence of Sn(II) ions. However, it is challenging to directly determine the Sn speciation and oxidation state within commercially available toothpaste products due to the low weight loading of SnF 2 (0.454 wt% SnF 2 , 0.34 wt% Sn) and the amorphous, semi-solid nature of the toothpaste. Here, we show that dynamic nuclear polarization (DNP) enables 119 Sn solid-state NMR experiments that can probe the Sn speciation within commercially available toothpaste. Solid-state NMR experiments on SnF 2 and SnF 4 show that 19 F isotropic chemical shift and 119 Sn chemical shift anisotropy (CSA) are highly sensitive to the Sn oxidation state. DNP-enhanced 119 Sn magic-angle turning (MAT) 2D NMR spectra of toothpastes resolve Sn(II) and Sn(IV) by their 119 Sn chemical shift tensor parameters. Fits of DNP-enhanced 1D 1 H → 119 Sn solid-state NMR spectra allow the populations of Sn(II) and Sn(IV) within the toothpastes to be estimated. This analysis reveals that three of the four commercially available toothpastes contained at least 80% Sn(II), whereas one of the toothpaste contained a significantly higher amount of Sn(IV). Oral health is highly important for a person’s overall physical health and well-being [1] , [2] , [3] , [4] . Toothpaste is the most commonly used dental hygiene product to maintain oral health by preventing and protecting against oral diseases, such as caries (i.e., cavities/tooth decay) and gingivitis (i.e., gum disease) [5] . Within commercial toothpastes, fluoride is the most effective active ingredient to prevent caries/cavities [1] , [5] , [6] , [7] , [8] , [9] , [10] . Stannous fluoride (SnF 2 ), one of three fluoride sources recognized by the United State Food and Drug Administration, has been used since the 1950’s as an effective way to deliver fluoride ions to tooth enamel and dentin [11] , [12] , [13] , [14] . However, early toothpastes exhibited challenges associated with the stability of SnF 2 and its compatibility with other ingredients [14] , [15] , [16] , [17] . Fortunately, advances in formulation technologies over the last couple decades have resulted in toothpastes with reportedly stable SnF 2 [14] , [17] , [18] , [19] , [20] , [21] . The use of SnF 2 as a fluoride source is highly appealing because SnF 2 has been shown to be an effective antimicrobial agent; antimicrobial agents help reduce gingivitis and plaque formation [15] , [21] , [22] , [23] , [24] , [25] , [26] , [27] , [28] , [29] , [30] . The antimicrobial properties associated with SnF 2 in toothpaste is thought to arise from the presence of Sn cations with an oxidation state of +2 [Sn(II)] [21] , [23] , [31] , [32] , [33] . Therefore, it is important that the majority of Sn within commercially available toothpaste maintains the +2 oxidation state [21] , [23] , [31] , [32] , [33] . However, Sn(II) cations are generally unstable and will readily oxidize to the more stable Sn(IV) cations upon air exposure. Commercial toothpaste formulations have various additives designed to stabilize Sn(II) compounds within the formulation. But, it is challenging to directly determine the Sn speciation and oxidation state within commercially available toothpaste due to the low weight loading of SnF 2 (0.454 wt%, 0.34 wt% Sn) and the amorphous semi-solid nature of the toothpaste. In 2019, Myers and co-workers used Sn K-edge X-ray Absorption Near Edge Spectroscopy (XANES) to determine that Colgate Total SF contains approximately 85% of its tin in the Sn(II) oxidation state [17] . More recently, Desmau and co-workers probed the Sn oxidation state within commercially available toothpastes via Sn K-edge XAS [34] . In both reports, the relative populations of Sn(II) and Sn(IV) species were estimated by fitting the experimental XAS spectra with XAS spectra of Sn(II) and Sn(IV) standards. However, XAS provides only a partial picture of chemical structure, and energy differences of the Sn(II) and Sn(IV) Sn K-edge spectral features are relatively small (~2.5 eV) and overlapping. Magic-angle spinning (MAS) solid-state NMR spectroscopy is a powerful technique to determine structure within crystalline and amorphous solids. Sn possess three NMR active isotopes ( 115 Sn, 117 Sn, and 119 Sn), with 119 Sn generally being the preferred nucleus to probe because it has the largest gyromagnetic ratio (2.7 times lower than 1 H) and natural isotopic abundance (8.59%). 119 Sn exhibits a large isotropic chemical shift range that is highly dependent on the local electronic structure surrounding the Sn atom [35] , [36] , [37] , [38] , [39] , [40] , [41] , [42] , [43] , [44] , [45] . In addition, the magnitude of the chemical shift anisotropy (CSA) is highly dependent on the symmetry at the Sn atom; asymmetric Sn coordination environments yield large CSA and broad NMR spectra. The magnitude of CSA is often quantified with the span (Ω) which is calculated from the difference of the largest and smallest principal components of the magnetic shielding tensor (Ω = σ 33 – σ 11 ) or the chemical shift tensor (Ω = δ 11 – δ 33 ) [46] , [47] . In general, Sn(IV) adopts a much more symmetric structure than its corresponding Sn(II) analogs and likely has larger differences in energy between occupied and unoccupied orbitals. For these reasons, Sn(IV) compounds tend to have smaller CSA than Sn(II) compounds [40] , [48] , [49] . For example, 119 Sn NMR spectra of Sn(IV) systems typically reveal spans of 0–200 ppm [36] , [40] , [48] , [49] , [50] , [51] , [52] , [53] , [54] , [55] , whereas for Sn(II) compounds, the span is often between ~ 700–1000 ppm and can be upwards of ~4000 ppm [39] , [40] , [41] , [48] , [49] , [53] , [56] , [57] , [58] , [59] , [60] , [61] , [62] . We note that there have been a few reports of Sn(IV) or Sn(II) exhibiting relatively large or small spans, respectively, due to either distorted or highly symmetric coordination environments, respectively [49] , [62] , [63] , [64] , [65] . Unfortunately, conventional room temperature 119 Sn MAS NMR spectroscopy of commercial toothpaste is not practically feasible due to the low weight loading of Sn within commercial toothpastes (~ 0.34 wt% Sn). In addition, the semi-solid nature of toothpaste will likely result in molecular mobility that causes the full or partial averaging of the 119 Sn CSA at room temperature. Additionally, solution 119 Sn NMR is also hindered by the semi-solid nature of toothpaste. Here, we apply cryogenic MAS dynamic nuclear polarization (DNP) [66] , [67] , [68] , [69] to enhance 119 Sn solid-state NMR signals of frozen toothpastes by one to two orders of magnitude, allowing 1D 119 Sn solid-state NMR spectra to be obtained in minutes from dilute commercial toothpaste formulations. Conventional room temperature solution and solid-state NMR experiments are performed on SnF 2 and SnF 4 . In a MAS DNP experiment, microwave irradiation is used to saturate electron paramagnetic resonance transitions, resulting in the subsequent transfer of electron spin polarization from stable free radicals to the 1 H spins of the solvent matrix and/or analyte [66] , [67] , [68] . Toothpastes typically contain high amounts of water and/or glycerol; water/glycerol mixtures have been shown to be an ideal matrix for MAS DNP experiments [66] . We note that the use of DNP to enable the acquisition of 119 Sn solid-state NMR spectra of dilute Sn(IV) species has been previously demonstrated [55] , [70] , [71] , [72] , [73] , [74] , [75] . To enable DNP experiments the AMUPol biradical [76] was directly dissolved in the toothpaste formulation. The DNP experiments were performed at ca. 110 K on frozen toothpaste. Freezing the toothpaste is beneficial because it eliminates any molecular motion, allowing measurement of 119 Sn CSA and enables 1 H- 119 Sn cross-polarization (CP) to transfer the DNP-enhanced 1 H polarization to 119 Sn nuclei. The 119 Sn CSA is shown to be a sensitive probe of the Sn oxidation state and from fits of the 1D 119 Sn solid-state NMR spectra the relative amounts of Sn(II) and Sn(IV) within the formulation can be estimated. Sn(II) and Sn(IV) Fluoride— 19 F and 119 Sn Chemical Shifts and Sample Purity Analysis. We first performed room temperature 19 F and 119 Sn solid-state NMR spectroscopy on SnF 2 and SnF 4 to determine chemical shift tensor parameters of Sn in the II or IV oxidation state, respectively. SnF 4 features Sn in the more stable IV oxidation state, with each Sn atom residing in a symmetric octahedral environment coordinated by 6 F atoms (Fig. 1A ) [77] . Consequently, no spinning sidebands are observed in the 119 Sn solid-state NMR spectrum of SnF 4 recorded with a 25 kHz MAS frequency, indicating Ω is less than 170 ppm (Fig. 1B , upper). Note throughout this entire manuscript, the Herzfeld-Berger convention is used to report the CSA [46] , [47] . α-SnF 2 contains Sn in the less stable, II oxidation state and there are two unique Sn sites in asymmetric environments that are coordinated by three or five F atoms (Fig. 1A ) [78] . 1D 119 Sn NMR spectra of SnF 2 were recorded for samples purchased from two different suppliers. The 119 Sn NMR spectrum of SnF 2 (supplier b ) reveals two isotropic 119 Sn NMR signals with δ iso = –948 ppm or –1023 ppm and Ω = 990 ppm or 930 ppm, respectively (skew = κ = 1.0 in both cases; Fig. 2B , lower). The 119 Sn NMR spectrum of SnF 2 (supplier b ) is consistent with prior reports and the structure determined from single-crystal X-ray diffraction [59] , [79] . On the other hand, the sample from supplier a shows additional 19 F and 119 Sn NMR signals. These additional NMR signals are attributed to Sn(IV) fluoride impurities because the observed 19 F chemical shifts, 119 Sn CSA, and correlations observed in the 2D 19 F{ 119 Sn} J -HMQC spectrum are similar to those observed for SnF 4 (Fig. 1B and 2 and Supplementary Fig. 2 ). We note that the 19 F chemical shift of tin fluoride materials appear to be sensitive to the Sn oxidation state; SnF 2 and SnF 4 exhibit a Δ δ iso ( 19 F) of 100 ppm (Fig. 2A ). Fig. 1: Crystal structures, 119 Sn solid-state NMR spectra and 19 F{ 119 Sn} J-HMQC solid-state NMR spectra. A Crystal structures of (left) SnF 4 and (right) SnF 2 [77] , [78] . B 1D 119 Sn spin echo NMR spectra of (upper to lower) SnF 4 , SnF 2 from supplier a and SnF 2 from supplier b recorded with a 25 kHz MAS frequency. An analytical simulation of the 119 Sn solid-state NMR spectrum of SnF 2 is shown below with fits of sideband intensities shown for the SnF 3 and SnF 5 sites (solid green and orange peaks, respectively). Estimated and fitted chemical shift tensor spans (Ω) are indicated. C 2D 19 F{ 119 Sn} J -HMQC NMR spectra of SnF 2 from (upper) supplier a and (lower) supplier b. Spectra were recorded with J -evolution times (τ J ) of 100 μs. Asterisks (*) indicate spinning sidebands. Full size image Fig. 2: Solution and solid-state 19 F NMR spectra and solution 19 F{ 119 Sn} HSQC NMR spectrum. A 19 F spin echo NMR spectra of (upper to lower) the model toothpaste, SnF 4 and SnF 2 (supplier b ) recorded in either (upper) solution or (lower two) the solid-state. Integrated peak intensities are indicated on the solution 19 F NMR spectrum (red). Asterisks indicate spinning sidebands. B Modified 19 F{ 119 Sn} J -HSQC pulse sequence that allows for evolution of the 19 F- 119 Sn J -coupling during the 119 Sn t 1 -evolution period. τ J denotes time periods for evolution of heteronuclear J -couplings. Note the absence of the 19 F π-pulse in the center of the t 1 -evolution period. C Solution 2D 19 F{ 119 Sn} J -HSQC NMR spectrum of the model toothpaste acquired with the pulse sequence shown in ( B ). Splittings due to 19 F- 119 Sn one-bond J -couplings ( 1 J ) are indicated. Full size image Periodic plane-wave density-functional theory (DFT) calculations utilizing the gauge-including projector-augmented wave (GIPAW) method predicts that the 119 Sn isotropic shielding (σ iso ) and Ω of two Sn species in SnF 2 differ by 76 and 68 ppm, respectively, and that the most shielded (i.e., most negatively shifted) Sn site exhibits the smaller Ω (Table S1 ). The most shielded Sn site is coordinated by 5 F atoms. The predicted difference in σ iso /δ iso and Ω is in excellent agreement with that observed experimentally, where the δ iso and Ω differ by ca . 75 and 60 ppm, respectively. Therefore, we assign the two 119 Sn NMR signals with δ iso = –948 ppm (Ω = 990 ppm) or –1023 ppm (Ω = 930 ppm) to Sn coordinated by three or five F atoms, respectively. We note that while the difference in the DFT calculated Ω is in excellent agreement with that observed experimentally, the magnitude of the DFT calculated Ω is smaller (Table S1 ). GIPAW calculations do not account for relativistic effects, which are likely needed to accurately calculate 119 Sn CS tensors [80] , [81] . GIPAW calculated 19 F chemical shielding values are in reasonable agreement with experiment (Supplementary Fig. 1 ). The calculations predict that SnF 2 should have 19 F chemical shifts which are approximately 100 ppm more positive than those of SnF 4 . The 119 Sn NMR spectrum of SnF 4 shows multiple 119 Sn NMR signals that all exhibit small CSA, revealing that this SnF 4 sample contains impurities (Fig. 1B , upper). A 1D 19 F spin echo NMR spectrum reveals three NMR signals between ca . –120 ppm to –160 ppm (Fig. 2A ); but, only two 19 F NMR signals are expected for the terminal and bridging F atoms in a 1:2 ratio, respectively (Fig. 1A ). We recorded a 2D 19 F{ 119 Sn} J -HMQC NMR spectrum to better probe the SnF 4 species from the impurities within this material (see Supplementary Material , Supplementary Fig. 1 ). Only the 119 Sn NMR signals at ca . –750 ppm and –785 ppm show correlations to two unique 19 F NMR signals at ca . 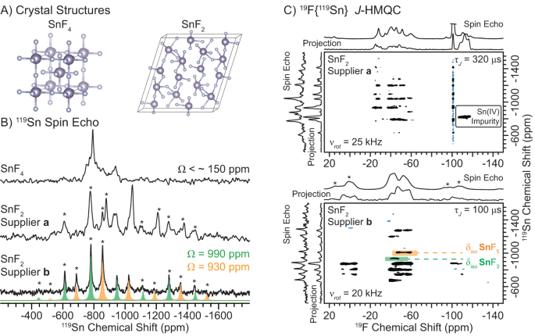Fig. 1: Crystal structures,119Sn solid-state NMR spectra and19F{119Sn} J-HMQC solid-state NMR spectra. ACrystal structures of (left) SnF4and (right) SnF277,78.B1D119Sn spin echo NMR spectra of (upper to lower) SnF4, SnF2from supplieraand SnF2from supplierbrecorded with a 25 kHz MAS frequency. An analytical simulation of the119Sn solid-state NMR spectrum of SnF2is shown below with fits of sideband intensities shown for the SnF3and SnF5sites (solid green and orange peaks, respectively). Estimated and fitted chemical shift tensor spans (Ω) are indicated.C2D19F{119Sn}J-HMQC NMR spectra of SnF2from (upper) supplieraand (lower) supplierb.Spectra were recorded withJ-evolution times (τJ) of 100 μs. Asterisks (*) indicate spinning sidebands. –130 ppm and –150 ppm; the difference in the 19 F isotropic chemical shift [Δ δ iso ( 19 F)] for the latter two sites agrees with that predicted by GIPAW DFT calculations (Δ σ iso ( 19 F) = 26 ppm, Supplementary Table 1 ). Therefore, both 119 Sn NMR signals at ca . –750 ppm and –785 ppm could plausibly be ascribed to SnF 4 . However, we tentatively assign the −785 ppm 119 Sn NMR signal to SnF 4 based on the much larger signal intensity observed in the 1D 119 Sn spin echo NMR spectrum and the 19 F chemical shifts observed in the 1D 19 F spin echo NMR spectrum (Fig. 1B and S1 ). We suspect that the other unassigned signals are derived from impurities, such as hydrated phases or other polymorphic forms of SnF 4 . 2D 19 F{ 119 Sn} J -HMQC NMR spectra of SnF 2 from supplier b reveals the expected correlations between all 19 F and 119 Sn NMR signals associated with SnF 2 (Fig. 1C , lower and Supplementary Fig. 3 ). The 2D 19 F{ 119 Sn} J -HMQC NMR spectrum of SnF 2 from supplier a reveals additional correlations between different 19 F and 119 Sn NMR signals that were not observed for SnF 2 from supplier b (Fig. 1C , upper). Notably, two unique sets of 19 F NMR signals of SnF 2 from supplier a resonate at significantly lower δ iso ( 19 F) than expected for SnF 2 ; the δ iso ( 19 F) is near that observed for SnF 4 (Supplementary Fig. 2 ). The lowest frequency 19 F NMR signal correlates with a 119 Sn that exhibits no observable CSA with a 25 kHz MAS frequency. Based on the low frequency 19 F NMR signal and small 119 Sn CSA, we assign these NMR signals to Sn(IV) fluoride impurities. We note that the observed 19 F and 119 Sn NMR signals are different than those assigned to SnF 4 . In summary, SnF 2 exhibits a significantly larger 119 Sn CSA than SnF 4 , illustrating that the 119 Sn CSA is a good probe of the Sn oxidation state, consistent with prior literature. Additionally, the 19 F chemical shifts for SnF 2 are much more positive than those for SnF 4 , suggesting that 19 F NMR can also provide insight into the Sn oxidation state. Interestingly, impurities in the SnF 2 and SnF 4 samples from supplier a were detected in 1D 19 F and 119 Sn NMR spectra. Notably, a 2D 19 F{ 119 Sn} J -HMQC spectrum of SnF 2 from supplier a revealed an Sn(IV) fluoride impurity. The observation of an Sn(IV)-based impurity is important because SnF 2 -based toothpastes rely on maximum Sn(II) availability for optimal performance. Impure SnF 2 starting materials will lead to a less effective toothpaste. 19 F and 119 Sn MAS solid-state NMR spectroscopies are good tools to determine the purity of tin fluoride materials, which may be used as precursors in toothpaste products. Solution 19 F and 119 Sn NMR Spectroscopy. We performed room temperature solution 19 F and 119 Sn NMR spectroscopy experiments on a model toothpaste to initially probe all Sn and F atoms before studying commercially available toothpastes with DNP-enhanced 119 Sn NMR spectroscopy. The model toothpaste consisted of ca . 2 wt% SnF 2 in a 1:2 mixture of D 2 O:glycerol d-8 ; the solution was prepared ca . 1 month before running NMR experiments. The use of SnF 2 in D 2 O:glycerol d-8 makes this a simplified version of most SnF 2 -based toothpastes, allowing for an easier assessment of the Sn speciation before studying more complex commercial toothpaste formulations. We note that the solution 19 F and 119 Sn NMR experiments suggest that the majority of F atoms are dissociated from Sn. As discussed in more detail below, we assume that only Sn atoms fully dissociated from F will be primarily observed in the DNP-enhanced 119 Sn solid-state NMR spectra because we lack the capability to decouple 19 F. The sizeable 19 F heteronuclear couplings for F coordinated tin ions could lead to reduced 119 Sn homogeneous transverse relaxation time constants ( T 2 ’) and low 119 Sn CPMG NMR signal intensities. A 1D 19 F solution NMR spectrum of the model toothpaste reveals primarily two 19 F NMR signals at –88.3 ppm and –157.4 ppm (Fig. 2A ). The broad hump from –150 ppm to –200 ppm is a probe background 19 F NMR signal (Supplementary Fig. 4 ). Closer examination of the –157.4 ppm 19 F NMR signal reveals three set of doublets centered around the isotropic NMR signal which correspond to 1-bond J -couplings of 19 F- 119 Sn (1571 Hz), 19 F- 117 Sn (1505 Hz) and 19 F- 115 Sn (1385 Hz) ( 1 J ; Fig. 2C , upper and Supplementary Fig. 4 ). The integral of each doublet matches with the corresponding Sn isotopic abundances and the J -couplings scale with the gyromagnetic ratios of the tin isotopes. We recorded a 2D 19 F{ 119 Sn} J -HMQC solution NMR spectrum to probe all F atoms bonded to Sn (Supplementary Fig. 5 ). Only the 19 F NMR signals near –155 ppm were observed in the 2D J -HMQC NMR spectrum. Therefore, we assign the 19 F NMR signal at –90 ppm to free fluoride ions. Integration of the 19 F NMR signals reveals that at least ca . 92% of F is present as ions within the D 2 O/glycerol d-8 mixture (Fig. 2A ). We note that the population of solvated F ions is likely even higher as the 19 F transmitter was on resonance with the F -Sn 19 F NMR signal and due to overlap of the –157.4 ppm signal with the probe background 19 F NMR signals (see Methods). The 19 F NMR signal assigned to an F -Sn species resonates at a similar shift as was observed for SnF 4 (Fig. 2A ). To confirm the origin of the –157.4 ppm 19 F NMR signal we recorded a 2D 19 F{ 119 Sn} J -HSQC solution NMR spectrum using the modified pulse sequence shown in Fig. 2B . The modified pulse sequence does not have a central refocusing (π) pulse applied to the 19 F spins during 119 Sn t 1 evolution, which causes evolution of 19 F- 119 Sn J -couplings and 119 Sn chemical shifts in the indirect dimension, resulting in a multiplet dependent on the number of attached F atoms to Sn. The modified 2D 19 F{ 119 Sn} J -HSQC solution NMR spectrum reveals a septet like pattern in the 119 Sn dimension and a doublet in the 19 F dimension ( 119 Sn decoupling was not performed during acquisition, Fig. 2C ). Note the central line of the septet pattern is absent because the central line of the multiplet arises from 119 Sn spins coupled to 3 19 F spin-up and 3 19 F spin-down leading to an effective J -coupling of 0 Hz. The observed 119 Sn septet matches exactly to that of a numerical simulation for Sn attached to six F atoms; the three doublets exhibit splittings at 2, 4, or 6 times 1 J Sn-F and the intensities are consistent with an AX 6 spin system determined from a modified Pascal triangle [82] . Therefore, the 19 F NMR signal at –157.4 ppm is assigned to the (SnF 6 ) −2 anions. In summary, integration of the 1D 19 F solution NMR spectrum suggests at most ca . 8% of F is directly bonded to Sn (Fig. 2A ). However, assuming that the two 19 F NMR signals correspond to free fluoride anions (F – ) and (SnF 6 ) –2 , then only ca . 2% of Sn within the model toothpaste contains F bonds, consistent with a 1D 119 Sn solution NMR spectrum that does not show appreciable amounts of Sn -F species (Supplementary Fig. 6 ). This observation is important because it implies essentially all Sn atoms are observable in the DNP 119 Sn solid-state NMR experiments. Sn species exhibiting F bonds would exhibit significant 119 Sn NMR signal attenuation in DNP solid-state NMR due to large 19 F- 119 Sn dipolar couplings that will not be effectively averaged in the absence of 19 F heteronuclear decoupling. Dynamic Nuclear Polarization 119 Sn Solid-State NMR Spectroscopy. We performed dynamic nuclear polarization (DNP) enhanced 119 Sn solid-state NMR spectroscopy on the model toothpaste, a commercially available preventative gel ( pg1 ) and four commercially available toothpastes ( t1 - t4 ). The weight loadings of SnF 2 in the model toothpaste, pg1 and t1 - t4 are ca . 2 wt%, 0.40 wt% or 0.454 wt%, corresponding to absolute Sn loadings of ca . 1.5 wt%, 0.30 wt% or 0.34 wt%, respectively. 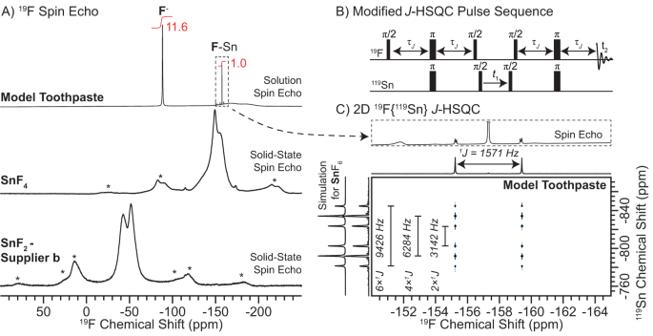Fig. 2: Solution and solid-state19F NMR spectra and solution19F{119Sn} HSQC NMR spectrum. A19F spin echo NMR spectra of (upper to lower) the model toothpaste, SnF4and SnF2(supplierb) recorded in either (upper) solution or (lower two) the solid-state. Integrated peak intensities are indicated on the solution19F NMR spectrum (red). Asterisks indicate spinning sidebands.BModified19F{119Sn}J-HSQC pulse sequence that allows for evolution of the19F-119SnJ-coupling during the119Snt1-evolution period. τJdenotes time periods for evolution of heteronuclearJ-couplings. Note the absence of the19F π-pulse in the center of thet1-evolution period.CSolution 2D19F{119Sn}J-HSQC NMR spectrum of the model toothpaste acquired with the pulse sequence shown in (B). Splittings due to19F-119Sn one-bondJ-couplings (1J) are indicated. pg1 contains primarily glycerol, similar to the model toothpaste (glycerol and water, Supplementary Table 2 ). t1 and t3 are glycerol-based, while t2 and t4 are water and glycerol and/or sorbitol-based. In addition the toothpastes contain other ingredients, such as abrasives (Table S2 ). t4 included SnCl 2 as an SnF 2 stabilizer. Samples were prepared for DNP experiments by directly dissolving the AMUPol biradical at a final concentration of 11 mM within the toothpastes (see Methods ). For the model toothpaste, H 2 O was added to increase DNP enhancements (10:30:60 ratio of H 2 O:D 2 O:gylcerol d-8 ). All DNP experiments were performed immediately after biradical addition. Prolonged storage of the DNP samples in a –20 °C freezer for days resulted in no DNP enhancements, likely due to reduction of the nitroxide biradical caused by conversion of Sn(II) to Sn(IV). In the absence of dissolved SnF 2 , the nitroxide biradical water glycerol solutions retain their DNP enhancements after months of storage in a freezer, consistent with reaction of Sn(II) with the nitroxide radicals causing the loss in DNP enhancements. 1 H → 13 C cross-polarization magic-angle spinning (CPMAS) DNP enhancements (ε) of the model toothpaste and pg1 were ca . 84 and 105, respectively (Fig. 3A and Supplementary Fig. 7 ). This means that acquisition of solid-state NMR spectra with the same signal-to-noise (SNR) ratio would take more than a thousand times longer to acquire without MW irradiation (i.e., no DNP). The DNP enhancement (ε) measured with 1 H → 119 Sn CP-CPMG experiments was estimated to be between 12–45 for the model toothpaste and t1 - t4 (Fig. 3B and Supplementary Fig. 8 ). However, a 119 Sn NMR spectrum could not be recorded without MW irradiation in a reasonable amount of time ( ca . 1 h). Therefore, we are likely under-estimating the 119 Sn DNP enhancements. The 119 Sn DNP enhancements are likely similar to those measured for 13 C since in both 119 Sn and 13 C cross-polarization NMR experiments, the magnetization is derived from the same bath of 1 H spins. The high DNP enhancements enables the acquisition of 2D 1 H- 119 Sn CP heteronuclear correlation (HETCOR) and magic-angle turning (MAT) NMR spectra of all samples. Fig. 3: DNP-enhanced 13 C and 119 Sn solid-state NMR spectra. Comparison of ( A ) 1 H → 13 C CPMAS and ( B ) 1 H → 119 Sn CP-CPMG NMR spectra of the model toothpaste recorded (black) with or (red) without microwave (MW) irradiation. The DNP enhancements (ε) are given in the figure. # denotes the truncated glycerol signal. DNP-enhanced ( C ) 1 H → 13 C and ( D ) 1 H → 119 Sn 2D CP-HETCOR NMR spectra of the model toothpaste. Spectra were recorded with a 10 kHz MAS frequency, eDUMBO 1–22 1 H homonuclear decoupling during 1 H indirect dimension evolution time, and CPMG detection of 119 Sn. The orange band illustrates that the same 1 H chemical shift is present in both 1 H NMR spectra. CP contact times (τ CP ) and total experiment times are indicated. Asterisks denote quadrature artifacts that occur at 1 H transmitter frequency. Full size image A 2D 1 H → 13 C CP-HETCOR NMR spectrum of the model toothpaste reveals correlations between the -O H 1 H NMR signals of glycerol or H 2 O and the 13 C NMR signals of glycerol (Fig. 3C ). The glycerol C H x 1 H NMR signals were not observed as the glycerol was fully deuterated. A 2D 1 H → 13 C CP-HETCOR NMR spectrum of preventative gel 1 reveals the expected correlations between all the 1 H and 13 C NMR signals of the CH x and -OH groups of the glycerol solvent (Supplementary Fig. 9A ). Interestingly, 2D 1 H → 119 Sn CP-CPMG HETCOR NMR spectra of the model toothpaste and pg1 both display correlations between all 1 H NMR signals observed in the 2D 1 H → 13 C CP-HETCOR NMR spectra with a broad 119 Sn NMR signal (Fig. 3D and Supplementary Fig. 9B ). The observed 1 H- 119 Sn correlations reveal that the Sn is present as ions that are likely solvated by H 2 O and/or glycerol. The interaction between Sn(II) and glycerol was also observed in liquid chromatography mass spectrometry (LCMS) experiments (Supplementary Fig. 10 ). 1D 1 H → 119 Sn CP-CPMG NMR spectra of all samples were acquired with multiple 119 Sn transmitter offsets (VOCS acquisition [83] , [84] ) due to the large breadth of the 119 Sn NMR signals and relatively low 119 Sn NMR excitation bandwidth (Supplementary Fig. 11 ). The 1D 1 H → 119 Sn CP-CPMG NMR spectra of the model toothpaste and pg1 reveal primarily a broad 119 Sn NMR signal ca . 1500 ppm in breadth, a larger range than was observed for SnF 2 ( ca . 1000 ppm). Likewise, the 1D 1 H → 119 Sn CP-CPMG NMR spectra of t1 - t4 reveal broad 119 Sn NMR signals that cover a range of ca . 1000–1500 ppm in addition to sharper 119 Sn NMR features. The broad 119 Sn NMR signals likely correspond to Sn(II) species whereas the sharper features likely correspond to Sn(IV). However, identification of Sn(II) and Sn(IV) species is fairly ambiguous from the 1D NMR spectra alone. The 1D 119 Sn MAS solid-state NMR spectra are likely broad and featureless because of the presence of isotropic chemical shift distributions, which are typical of disordered and amorphous systems. There is probably a distribution in the number of water, hydroxide, and glycerol (or glyceroxide) molecules coordinated to each tin ion. To resolve Sn(II) from Sn(IV) species based on their CSA, we recorded DNP-enhanced 2D 119 Sn adiabatic magic angle turning (aMAT) NMR spectra of all samples (Fig. 4 and S12 – S15 ) [85] , [86] , [87] , [88] . These 2D NMR experiments required only ca . 6 h for the model toothpaste (Sn loading ~ 1.5 wt%) and ca . 16–17 h for pg1 and t1 - t4 (Sn loading = 0.3 or 0.34 wt%, respectively). In a MAT NMR experiment, an isotropic NMR spectrum free of spinning sidebands (indirect dimension) is correlated with its corresponding anisotropic MAS NMR spectrum (direct dimension). Therefore, the anisotropic NMR spectra extracted at specific isotropic chemical shifts (δ iso ) can be easily fit to determine the span (Ω) and skew (κ) because the δ iso is known. Fig. 4: DNP-enhanced 119 Sn aMAT NMR spectra. 2D 119 Sn aMAT NMR spectra of ( A ) the model toothpaste and ( C ) t1 acquired with a 10 kHz MAS frequency, 1 H → 119 Sn CP at the start of the experiment, and CPMG for 119 Sn detection. B , D 119 Sn solid-state NMR spectra extracted from the 2D aMAT NMR spectra at the indicated 119 Sn isotropic chemical shifts (δ iso ). Analytically simulated spectra are shown (colored) below the (black) experimental MAS spectra. The values of the isotropic chemical shift (δ iso ), span (Ω) and skew (κ) used in the analytical simulations are indicated next to each row. Full size image 2D 119 Sn aMAT NMR spectra of the model toothpaste and pg1 are near identical and reveal broad isotropic 119 Sn NMR spectra in the region of ca . –600 to –1000 ppm (Fig. 4A and S12A ). The broad isotropic 119 Sn NMR spectra illustrate that there are large distributions in the 119 Sn δ iso , likely due to differences in the Sn ion coordination from the solvent matrix. We note that the center of the isotropic 119 Sn NMR spectrum of the model toothpaste appears at the same 119 Sn chemical shift observed in solution, however, the breadth of the signal is much narrower at room temperature due to dynamics of the Sn ions in solution (Supplementary Fig. 6 ). Anisotropic 119 Sn NMR spectra extracted from the isotropic 119 Sn dimension reveals primarily Sn sites with a Ω of ca . 1200 ppm and a κ of +0.7, which are assigned to Sn(II) species based on the large CSA (Fig. 4B and S12B ). However, anisotropic 119 Sn NMR spectra extracted at higher 119 Sn δ iso of ca . –750 ppm or –800 ppm to –600 ppm for the model toothpaste or pg1 , respectively, show an increased intensity for the isotropic (center band) NMR signals. An increase in intensity for the isotropic NMR signal reveals there are additional sites with spans of 150 ppm or less, but with identical 119 Sn isotropic chemical shift to sites that have a larger span; the small CSA sites should correspond to Sn(IV). Therefore, the 2D 119 Sn aMAT NMR spectra clearly reveal both Sn(II) and Sn(IV) sites based on their CSA. We note that the experimental anisotropic NMR spectra show distorted signal intensities at lower 119 Sn chemical shifts due to limited 119 Sn NMR excitation bandwidth. Nevertheless, Ω and κ can still be accurately determined by fitting the most intense spinning sidebands with the isotropic shift as a fixed constraint. DNP-enhanced 2D 119 Sn aMAT NMR spectra of t1, t2, and t3 are near identical and display three relatively sharp isotropic 119 Sn NMR signals at ca . –762 to –775 ppm, –732 to –744 ppm and –665 ppm, in addition to a broad isotropic 119 Sn NMR signal from ca . –500 to –600 ppm (Fig. 4C , S13A and S14A ). The relatively sharp 119 Sn NMR signals at ca . –762 to –775 ppm and –732 to –744 ppm clearly show intense isotropic 119 Sn NMR signals, which are assigned to Sn(IV) species based on the small Ω ( ca . 150 ppm; Fig. 4A , S13B and S14B ). There are additional weak sidebands associated with Sn that have spans on the order of ca . 1200 ppm, suggesting some Sn(II) species are present at these isotropic shifts. Anisotropic 119 Sn NMR spectra extracted at more positive 119 Sn δ iso of ca . –665 ppm and –600 ppm reveal significantly more intense broad 119 Sn NMR spectra with spans of ca . 1200 ppm (Fig. 4A , S13B and S14B ). At the lower 119 Sn δ iso of ca . –665 ppm, the isotropic NMR signal has increased signal intensity, consistent with additional small CSA sites (Ω ≈ 150–250 ppm). However, the more positively shifted isotropic 119 Sn NMR signals are clearly primarily associated with Sn(II) sites. We note that the isotropic 119 Sn NMR spectra are not representative of the Sn(II) and Sn(IV) populations due to differences in MAT efficiencies for high or low CSA sites, respectively. The similarities in the 2D 119 Sn aMAT spectra of t1 and t3 are not surprising because they are both primarily glycerol-based. However, the similarities between the MAT NMR spectrum of t2 with the MAT NMR spectra of t1 and t3 are interesting because t2 contains a significant amount of water in addition to glycerol. Interestingly, the 2D 119 Sn aMAT NMR spectrum of t4 is significantly different from that of t1 - t3 (Supplementary Fig. 15A ). As mentioned above, t4 contains primarily water and sorbitol (similar to t2 ), in addition to SnCl 2 as a SnF 2 stabilizer (Table S2 ). The isotropic 119 Sn NMR spectrum of t4 shows primarily three isotropic 119 Sn NMR signals at ca . –665 ppm, –550 ppm and –475 ppm (Supplementary Fig. 15B ). Similar 119 Sn isotropic NMR signals were observed for t1 - t3 , however, for t4 the 119 Sn isotropic NMR signals at ca . –665 and –550 ppm correspond to predominantly small CSA sites (Ω ~ 150–220 ppm; Supplementary Fig. 15B ). The 119 Sn isotropic NMR signal at ca . –475 ppm clearly shows sites with both large and small CSA (Ω ≈ 220 ppm and 1100 ppm). With knowledge of all 119 Sn chemical shift tensors, the 1D 1 H → 119 Sn CP-CPMG NMR spectra of all samples could be analytically simulated (Fig. 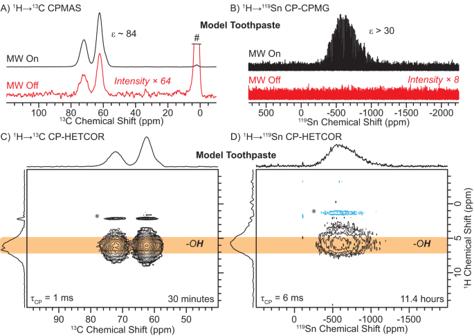Fig. 3: DNP-enhanced13C and119Sn solid-state NMR spectra. Comparison of (A)1H →13C CPMAS and (B)1H →119Sn CP-CPMG NMR spectra of the model toothpaste recorded (black) with or (red) without microwave (MW) irradiation. The DNP enhancements (ε) are given in the figure. # denotes the truncated glycerol signal. DNP-enhanced (C)1H →13C and (D)1H →119Sn 2D CP-HETCOR NMR spectra of the model toothpaste. Spectra were recorded with a 10 kHz MAS frequency, eDUMBO1–221H homonuclear decoupling during1H indirect dimension evolution time, and CPMG detection of119Sn. The orange band illustrates that the same1H chemical shift is present in both1H NMR spectra. CP contact times (τCP) and total experiment times are indicated. Asterisks denote quadrature artifacts that occur at1H transmitter frequency. 5 and Supplementary Table 3 ). The 2D 119 Sn aMAT NMR spectra revealed large distributions in the 119 Sn δ iso . Therefore, we fit the 1D 1 H → 119 Sn CP-CPMG NMR spectra to sites containing large amounts of Gaussian line broadening to represent the distributions in the isotropic chemical shifts. Fig. 5: DNP-enhanced MAS 1 H → 119 Sn CP-CPMG solid-state NMR spectra. (upper to lower) 1 H → 119 Sn CP-CPMG NMR spectra for the model toothpaste, pg1 , and t1 - t4 . Multiple CP-CPMG NMR spectra were recorded with different 119 Sn transmitter frequencies (i.e., VOCS style acquisition, Supplementary Fig. 11 ). All spectra were recorded with a 10 kHz MAS frequency and a sample temperature of approximately 110 K. Total fits are indicated by red dashed lines. Solid blue, brown, orange, and green peaks correspond to the individual sites used in fitting. Full size image The model toothpaste and pg1 display similar 1D 1 H → 119 Sn CP-CPMG NMR spectra, where the populations of Sn(II) were determined to be ca . 92 or 93%, respectively (Fig. 5 ). t1 - t3 also display similar 1D 1 H → 119 Sn CP-CPMG NMR spectra (Fig. 5 ). The populations of Sn(II) were determined to be ca . 80% for t1 and t3 and 90% for t2 . We also recorded a 1D 1 H → 119 Sn CP-CPMG NMR spectrum of t2 after allowing the toothpaste to dry out and exposing it to air over the course of 1 day (Fig. 5 ). Interestingly, the population of Sn(II) decreased from ca . 90 to 83%, resulting from oxidation of Sn(II) to Sn(IV) from O 2 in the atmosphere. This experiment was an important control that confirms our hypothesis that the 119 Sn NMR signals of Sn(IV) primarily have small spans, while those associated with Sn(II) have larger spans. Consistent with the differences observed in the 2D 119 Sn aMAT NMR spectrum, t4 displays a different 1D 1 H → 119 Sn CP-CPMG NMR spectrum with a significantly lower amount of Sn(II) ( ca . 68%; Fig. 5 ). We note that the relative populations of Sn(II) for t1 - t4 determined here are generally consistent with prior measurements made in Sn K-edge X-ray absorption studies [17] , [34] . There are three main mechanisms that can lead to inaccurate Sn(II) and Sn(IV) populations determined from the 1D 1 H → 119 Sn CP-CPMG NMR spectra: (1) differences in DNP enhancement, (2) difference in 1 H → 119 Sn CP dynamics, and (3) differences in 119 Sn refocused transverse relaxation time constants ( T 2 ’). DNP enhancements for Sn(II) and Sn(IV) should be identical since 2D 1 H → 119 Sn CP-HETCOR NMR spectra revealed that Sn is present as ions within the solvent matrix and 1 H spin diffusion should distribute the DNP enhanced 1 H polarization homogeneously across the frozen solution (Fig. 3D and Supplementary Fig. 9B ). 1 H → 119 Sn CP dynamics are likely similar for Sn(II) and Sn(IV) sites since they are both likely coordinated by water, hydroxide ions and/or glycerol molecules. However, 1 H → 119 Sn CP is likely less efficient for sites with high CSA because the CSA is comparable to or larger than the RF field used for the 119 Sn spin-lock pulse. From this perspective, the Sn(II) populations are likely a lower bound. To assess differences in 119 Sn T 2 ’, we investigated the effect that the number of CPMG echoes used during that acquisition of 1 H → 119 Sn CP-CPMG NMR spectra of the model toothpaste and t1 had on the determined Sn(II) and Sn(IV) populations (Supplementary Fig. 16 ). 1 H → 119 Sn CP-CPMG NMR spectra processed with 1 to 100 spin echoes in the CPMG train reveal near identical populations of Sn(II) and Sn(IV), confirming that the 119 Sn T 2 ’ must be similar for all species. The observation of similar 119 Sn T 2 ’ for all Sn species is also consistent with minimal Sn sites exhibiting F bonds, as those sites would exhibit a shorter 119 Sn T 2 ’. Therefore, analytical simulations of the 1 H → 119 Sn CP-CPMG NMR spectra likely reveal relatively accurate populations of Sn(II) and Sn(IV), where the population of Sn(II) should be taken as a lower bound due to differences in CP efficiencies. In conclusion, we applied dynamic nuclear polarization (DNP) enhanced 119 Sn solid-state NMR spectroscopy to determine the Sn oxidation state and speciation within commercially available SnF 2 -based toothpastes that contain loadings of less than 0.5 wt%. We first obtained room-temperature 19 F and 119 Sn solid-state NMR spectra of SnF 2 and SnF 4 . These experiments confirmed Sn(II) exhibits a near order of magnitude larger span than that of Sn(IV), consistent with prior literature. NMR studies of SnF 2 purchased from two different suppliers revealed a significant amount of Sn and F-based impurities in one of the samples. Notably, 2D 19 F{ 119 Sn} J -HMQC NMR spectra revealed that the impure SnF 2 sample contains Sn(IV) fluoride-based impurities. 19 F and 119 Sn solid-state NMR are good probes of the purity of SnF 2 precursors used in the production of toothpastes. Solution 19 F and 119 Sn NMR studies on a model toothpaste consisting of ca . 2 wt% SnF 2 in a 50:50 mixture of D 2 O:glycerol d-8 suggested that only ca . 2% of the dissolved Sn ions contain F bonds. DNP experiments of model and commercially available toothpastes were enabled by directly mixing the DNP polarizing agent (AMUPol biradical) within the toothpaste. Importantly, the sensitivity gains offered by DNP enabled detection of 119 Sn NMR signals from toothpastes with loadings of 0.34 wt% Sn. 2D 1 H → 13 C and 1 H → 119 Sn CP-HETCOR NMR spectra of the model toothpaste and pg1 suggested that all Sn is present as ions that are solvated by water, hydroxide anions and/or glycerol. 1D 1 H → 119 Sn CP-CPMG NMR spectra of all toothpastes revealed broad 119 Sn NMR spectra, with some additional sharper features. Acquisition of 2D 119 Sn magic-angle turning (MAT) NMR spectra of all samples allowed for the unambiguous identification of Sn(II) and Sn(IV) species based on their CSA. With knowledge of the 119 Sn chemical shift tensor parameters, 1D 1 H → 119 Sn CP-CPMG NMR spectra were fit to estimate the populations of Sn(II) and Sn(IV) within the toothpastes. Notably, three of the four commercially available toothpastes contained at least 80% Sn(II), whereas one of the toothpaste contained a significantly higher amount of Sn(IV). We have demonstrated that DNP-enhanced 119 Sn solid-state NMR spectroscopy is an ideal technique to probe the Sn speciation with commercially available toothpastes. The determination of the Sn(II) and Sn(IV) populations within commercially available toothpastes is important both to assess the quality of current formulations and to develop new and improved formulations. Increasing the amount of Sn(II) should increase the antimicrobial properties of SnF 2 -based toothpastes. We observed that both glycerol-based toothpastes ( t1 and t3 ) and toothpastes containing high amounts of water and glycerol ( t2 ) can exhibit high amounts of Sn(II) ( ca . 80–90%). However, the Sn(II) is readily oxidized to Sn(IV) after prolonged air-exposure. More detailed studies on the specific coordination of Sn and their interactions with other common toothpaste ingredients are on-going in our labs. By better understanding how common toothpaste ingredients interact with Sn, and specifically Sn(II), DNP-enhanced 119 Sn solid-state NMR spectroscopy will enable the rational design and development of next-generation SnF 2 -based toothpastes that exhibit increased Sn(II) availability and long-term oxidation stability. Samples of SnF 4 and SnF 2 (supplier a ) were purchased from Sigma Aldrich, Inc. SnF 2 supplier b corresponds to the SnF 2 that is used in commercial toothpaste products. AMUPol was purchased from CortecNet Inc. Glycerol- d 8 and D 2 O were purchased from Sigma-Aldrich Inc. All materials were used as received without further purification. Two different model toothpastes were prepared for solution NMR experiments and DNP solid-state NMR experiments, respectively. A micropipette was used to transfer the water-glycerol solutions. However, due to the high viscosity of the glycerol solutions, an analytical balance was used to weigh the amount of solution transferred to ensure that the desired volumes of water, glycerol and water-glycerol solutions were transferred. For the solution NMR experiments, a 2 wt% SnF 2 solution was prepared by dissolving 7.1 mg of SnF 2 in 347.6 mg of a 1:2 volume fraction solution of D 2 O:glycerol- d 8 . The solution was stored for 1 month at room temperature before running solution NMR experiments. The model toothpaste for DNP solid-state NMR experiments was prepared by first making approximately 200 μL (260 mg) of a stock solution of 10:30:60 volume fraction H 2 O:D 2 O:glycerol- d 8 . 2.2 mg of SnF 2 was weighed out and 107.9 mg of the stock H 2 O:D 2 O:glycerol- d 8 solution was added to give a final SnF 2 concentration of 2 wt%. The SnF 2 was allowed to dissolve over the course of approximately 2 h. This solution as then stored in a freezer until it was needed. To prepare samples for DNP experiments, a few mg of the AMUPol biradical were then weighed out in a glass vial and SnF 2 H 2 O:D 2 O:glycerol- d 8 stock solution was then added to obtain a final AMUPol concentration of 10 ± 2 mM. Approximately 20 μL of this solution was then transferred to a sapphire DNP rotor which was then capped with a silicone plug and a zirconia drive cap. The packed rotor was then transferred into the pre-cooled DNP probe within 20 min to limit oxidation of the Sn 2+ ions by reaction with AMUPol. AMUPol was used for DNP experiments because this radical gives high DNP enhancements and sensitivity gains at 9.4 T for water-glycerol based mixtures [66] . Samples of commercial toothpastes were prepared for DNP experiments by directly mixing the AMUPol biradical within the toothpastes to obtain a final AMUPol concentration of ca . 10 mM. A typical sample preparation of the commercial toothpastes for DNP consisted of weighing out the AMUPol biradical in a vial ( ca . 1.3–2.3 mg), adding the proper amount of toothpaste to reach a concentration of ca . 10 mM, and then vigorously stirring the toothpaste for ca . 10 min to ensure the radical was homogenously mixed throughout the toothpaste. The densities of the toothpastes were assumed to be ca . 1.3 g cm −3 . We note that samples of toothpastes 1 – 4 were taken from the middle of a fresh toothpaste tube, while preventative gel 1 was taken from the top of a fresh tube. During the mixing step, the vial was periodically held under a stream of warm water for short time periods (a maximum time of ca . 10 s) to decrease the viscosity of the toothpaste and facilitate better mixing and dissolution of the radical. Once the radical was homogenously mixed with the toothpaste, the sample was immediately packed into a 3.2 mm sapphire rotor. The sapphire rotor was sealed with a silicone soft plug and capped with a zirconia drive cap. All DNP samples were prepared immediately before performing NMR experiments. The maximum time it took to prepare the sample and insert the rotor into the spectrometer was ca . 20–30 min. We note that prolonged storage (1–2 weeks) of the prepared samples at ca . 0 °C gave no DNP enhancements due to reduction of the biradical, presumably caused by oxidation of Sn(II) to Sn(IV). Room temperature solution 19 F and 119 Sn solution NMR experiments were performed on the model toothpaste and recorded on a 9.4 T (ν 0 ( 1 H) = 400 MHz) Bruker standard-bore magnet equipped with a AVANCE NEO console and a liquid-N 2 cooled Bruker Prodigy HXY NMR probe. 19 F and 119 Sn chemical shifts were referenced to CCl 3 F and SnMe 4 , respectively, with D 2 O as the lock signal. The 19 F π/2 and π pulses were 15 and 30 μs in duration, corresponding to a 16.7 kHz radio frequency (RF) field. We note that the 19 F NMR spectrum was recorded with the 19 F transmitter on resonance with the SnF 6 −2 19 F NMR signal. The 19 F NMR signals of the free F ions were ca . 26 kHz away from the 19 F transmitter. The 19 F spin echo NMR spectrum was recorded with 100 μs delays on each side of the 19 F π pulse. The 19 F solution NMR spectra were acquired with different recycle delays to ensure that quantitative relative peak intensities were obtained. 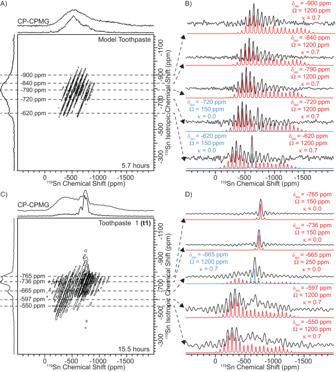Fig. 4: DNP-enhanced119Sn aMAT NMR spectra. 2D119Sn aMAT NMR spectra of (A) the model toothpaste and (C)t1acquired with a 10 kHz MAS frequency,1H →119Sn CP at the start of the experiment, and CPMG for119Sn detection.B,D119Sn solid-state NMR spectra extracted from the 2D aMAT NMR spectra at the indicated119Sn isotropic chemical shifts (δiso). Analytically simulated spectra are shown (colored) below the (black) experimental MAS spectra. The values of the isotropic chemical shift (δiso), span (Ω) and skew (κ) used in the analytical simulations are indicated next to each row. 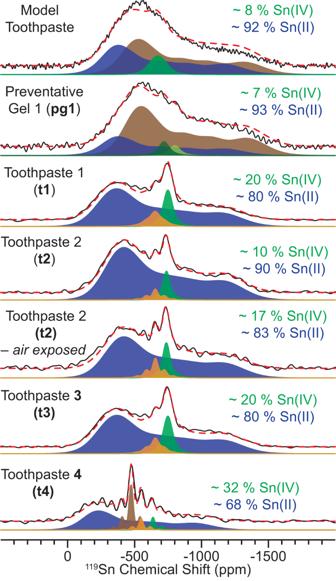Fig. 5: DNP-enhanced MAS1H →119Sn CP-CPMG solid-state NMR spectra. (upper to lower)1H →119Sn CP-CPMG NMR spectra for the model toothpaste,pg1, andt1-t4. Multiple CP-CPMG NMR spectra were recorded with different119Sn transmitter frequencies (i.e., VOCS style acquisition, Supplementary Fig.11). All spectra were recorded with a 10 kHz MAS frequency and a sample temperature of approximately 110 K. Total fits are indicated by red dashed lines. Solid blue, brown, orange, and green peaks correspond to the individual sites used in fitting. Recycle delays used for solution NMR experiments are given in Supplementary Table 4 . The 119 Sn π/2 and π pulses were 12.5 μs and 25 μs in duration, corresponding to a 20 kHz RF field. The 119 Sn spin echo NMR spectrum was recorded with 10 μs echo delays on each side of the 119 Sn π pulse. Room Temperature solid-state NMR spectroscopy experiments were performed with a 9.4 T (ν 0 ( 1 H) = 400 MHz) Bruker wide-bore magnet equipped with a Bruker Avance III HD console and a 2.5 mm HXY magic-angle spinning (MAS) NMR probe configured in triple resonance mode. We note that the 19 F and 119 Sn match was relatively poor ( ca . 30 and 60% for 19 F and 119 Sn, respectively) when tuned simultaneously to 19 F and 119 Sn on the 1 H and X channel, respectively. The magnetic field was referenced to 1% tetramethyl silane (TMS) in CDCl 3 with adamantane (δ( 1 H) = 1.71 ppm) as a secondary chemical shift reference. 19 F and 119 Sn chemical shifts were indirectly referenced to CCl 3 F and SnMe 4 , respectively, using the previously published IUPAC recommended relative NMR frequencies [89] . The 19 F π/2 and π pulses were 4 and 8 μs in duration, corresponding to a 62.5 kHz radio frequency (RF) field. The 119 Sn π/2 and π pulses were 3.5 and 7 μs in duration, corresponding to a 71 kHz RF field. 2D 19 F{ 119 Sn} J -based heteronuclear multiple quantum correlation ( J -HMQC) experiments were recorded with the arbitrary indirect dwell (AID) HMQC pulse sequence [88] . SPINAL-64 heteronuclear decoupling with a 50 kHz 19 F RF field was performed during the acquisition of 119 Sn NMR signals [90] . 119 Sn and 19 F solid-state NMR spectra were acquired at multiple MAS frequencies to confirm the assignment of isotropic and sideband NMR signals (Supplementary Fig. 17 ). DNP-enhanced solid-state NMR spectroscopy experiments were performed with a 9.4 T (ν 0 ( 1 H) = 400 MHz) Bruker wide-bore magnet equipped with a 263 GHz gyrotron, a Bruker AVANCE III console and a 3.2 mm HXY MAS DNP NMR probe [67] . MAS solid-state NMR experiments were performed with a sample temperature of ca. 110 K. The magnetic field was referenced to 1% TMS in CDCl 3 with the 1 H shift of the silicone soft plug (δ( 1 H) = 0.24 ppm) as a secondary chemical shift reference. The 1 H shift of the silicone soft plug was determined based on the 1 H shift of frozen tetrachloroethane (TCE, δ( 1 H) = 6.2 ppm). 13 C and 119 Sn shifts were indirectly referenced to SiMe 4 or SnMe 4 , respectively, using the previously published IUPAC recommended relative NMR frequencies [89] . All NMR spectra were initially processed and referenced with the Bruker Topspin 3.6.1 software. Carr-Purcell Meiboom-Gill (CPMG) echo trains were co-added using the NUTs NMR software (Acorn, Inc.). The 119 Sn solid-state NMR spectra were analytically fit using the open-source ssNake NMR software [91] . All experimental NMR parameters (MAS frequency, recycle delay (τ rec. delay ), number of scans, t 1 dwell (Δ t 1 ), t 1 TD points, t 1 acqusition time ( t 1 AQ), CP/ J -evolution durations (τ CP/ J -evolv. ) and total experimental times are given in Supplementary Table 4 . DNP NMR experiments were performed with the NMR probe configured in either HXY triple-resonance mode (tuned to 1 H- 119 Sn- 13 C) or HX double-resonance mode (tuned to 1 H- 119 Sn). In all probe configurations, the 1 H π/2 and π pulse lengths were 2.5 and 5 μs in duration, corresponding to a 100 kHz RF field. The 13 C π/2 and π pulse lengths were 4 and 8 μs in duration, corresponding to a 62.5 kHz RF field. In triple-resonance HXY mode, the 119 Sn π/2 and π pulse lengths were 4 and 8 μs in duration, corresponding to a 62.5 kHz RF field. In double-resonance HX mode, the 119 Sn π/2 and π pulse lengths were 3 and 6 μs in duration, corresponding to an 83.3 kHz RF field. 1 H → 13 C cross-polarization (CP) was achieved with a 10 kHz MAS frequency with simultaneous 1 H and 13 C spin-lock pulses with RF fields of ca . 62 kHz (ramped from 56–62 kHz) and 64 kHz, respectively. In triple-resonance HXY mode (10 kHz MAS frequency), 1 H → 119 Sn CP was achieved with simultaneous 1 H and 119 Sn spin-lock pulses with RF fields of ca . 72 kHz (ramped from 65–72 kHz) and 56 kHz, respectively. In double-resonance HX mode (10 kHz MAS frequency), 1 H → 119 Sn CP was achieved with simultaneous 1 H and 119 Sn spin-lock pulses with RF fields of ca . 76 kHz (ramped from 69 – 76 kHz) and 80 kHz, respectively. Optimization of the 1 H → 119 Sn CP contact time showed that 6 ms was optimal. All 119 Sn NMR spectra were acquired with CPMG detection to increase sensitivity. π/2 (1D NMR spectra of t1 – t4 ) or π (all other spectra) pulses were implemented in the CPMG trains [92] , [93] . 1D 1 H → 119 Sn CP-CPMG NMR spectra were acquired with multiple 119 Sn transmitter offsets due to the large breadth of the 119 Sn NMR spectra (i.e., VOCS style acquisition; Supplementary Fig. 11 ) [83] , [84] . 2D 1 H → 13 C and 1 H → 119 Sn CP-HETCOR NMR spectra were recorded with 100 kHz 1 H RF field of eDUMBO 1–22 homonuclear dipolar decoupling applied during the t 1 -evolution period [94] . Each pulse in the homonuclear dipolar decoupling train was 32 μs in duration. 2D 119 Sn adiabatic magic-angle turning (aMAT) NMR spectra were recorded with the published pulse sequences [85] , [86] , [87] , [88] . Frequency swept tanh/tan inversion pulses were 100 μs in duration (i.e., 1 rotor-cycle for a 10 kHz MAS frequency) with an ca . 90 kHz RF field, a 2 MHz sweep width and 400 points. All 119 Sn aMAT spectra were recorded with 1 H → 119 Sn CP at the start of the experiment and with the arbitrary indirect dwell (AID) t 1 acquisition mode to increase sensitivity [88] . 100 kHz 1 H RF field of SPINAL-64 heteronuclear decoupling was performed during the acquisition of 13 C and 119 Sn [90] .